LSD1 co-repressor Rcor2 orchestrates neurogenesis in the developing mouse brain Epigenetic regulatory complexes play key roles in the modulation of transcriptional regulation underlying neural stem cell (NSC) proliferation and progeny specification. How specific cofactors guide histone demethylase LSD1/KDM1A complex to regulate distinct NSC-related gene activation and repression in cortical neurogenesis remains unclear. Here we demonstrate that Rcor2, a co-repressor of LSD1, is mainly expressed in the central nervous system (CNS) and plays a key role in epigenetic regulation of cortical development. Depletion of Rcor2 results in reduced NPC proliferation, neuron population, neocortex thickness and brain size. We find that Rcor2 directly targets Dlx2 and Shh, and represses their expressions in developing neocortex. In addition, inhibition of Shh signals rescues the neurogenesis defects caused by Rcor2 depletion both in vivo and in vitro . Hence, our findings suggest that co-repressor Rcor2 is critical for cortical development by repressing Shh signalling pathway in dorsal telencephalon. Previous studies have defined neural stem cell (NSC) and Neural Progenitor Cell (NPC) populations in the developing neuroepithelium of the rodent neocortex with region-specific neuronal progenies generated at embryonic stages. Whereas cortical projection excitatory neurons derive from radial glial cells (RGCs) at the dorsal (pallial) telencephalon and migrate radially into the cortical plate, neocortical interneurons are generated in the ventral telencephalon, including the ganglionic eminences and the preoptic area (PoA), and migrate tangentially over long distances to reach the neocortex [1] , [2] , [3] , [4] , [5] , [6] , [7] , [8] . During embryonic brain development, a series of morphogens are involved in the establishment of patterning in the neuroepithelum, which provide specific environments to form different substructures of functional brain. Multiple studies exploring the mechanism of temporal and spatial regulation that lead to the remarkable cellular diversity of the mature neocortex have underlined the importance of organizing signals such as Sonic hedgehog (Shh), fibroblast growth factors, WNTs, and bone morphogenetic proteins, which provide positional information in body axes [7] , [9] , [10] , [11] , [12] , [13] , [14] . Among these signals, Shh expression is first observed in the mesendoderm and diencephalon between E8.5 and E9 during telencephalic development, which are then restricted to the Medial Ganglionic Eminence (MGE) and PoA by E9.5 and by E12.5, respectively, to pattern the ventral brain, while maintaining a very low activity in the developing dorsal cortex [15] , [16] , [17] , [18] , [19] . However, how Shh signal is controlled and restricted to the specific regions and how Shh regulates NSC/NPC proliferation and differentiation still remains poorly understood. Extensive studies have suggested that NSC differentiation and fate specification is regulated by a series of intrinsic and extrinsic signals. Although the mechanisms of regional restriction and fate determination of NSCs are not yet fully understood, it is becoming apparent that intrinsic epigenetic regulation is closely involved through DNA methylation, histone modification and non-coding RNA expression [20] , [21] , [22] , [23] , [24] , [25] , [26] . Histone demethylase LSD1, also known as KDM1A, is a key component of various protein complexes that contain transcription co-repressors, including Rcor1 (CoREST), BHC80, HDAC1/2, CtBP, BRAF35 and several zinc finger proteins [26] , [27] , [28] . As the first identified RCOR protein, Rcor1 is widely studied in various types of cells, playing important roles in mouse erythropoiesis [29] and neuronal or synaptic gene regulation by modifying chromatin configuration [30] , [31] , [32] , [33] . Sharing 70% sequence similarities with Rcor1, Rcor2 can form a protein complex with LSD1, to facilitate its demethylase activity on nucleosome in embryonic stem cells (ESCs) [34] . Furthermore, Rcor2 but not Rcor1 has been described as a Sox2 substitute to regulate ESC proliferation and promote the formation of induced pluripotent stem cells [34] . However, the in vivo function of Rcor2 in development is unknown. Here we demonstrate that Rcor2 is mainly expressed in the central nervous system (CNS) and affects NSC proliferation and neurogenesis during cortical development. We find that Rcor2 associating with LSD1 plays a determinant role in directly binding to Dlx2 and Shh promoter regions, to inhibit gene expression. The disruption of Shh, the direct regulation target of Rcor2 and upstream effector of Dlx2, rescues the neurogenesis defects caused by Rcor2 depletion, suggesting that Rcor2 plays a critical role of temporal and spatial regulation of gene expressions to safeguard cortical neurogenesis in brain development. Rcor2 is mainly expressed in the CNS To analyse Rcor2’s function and mechanism during development, Rcor2 gene-trapped mice (Rcor2 LacZ ) were used as described in detail methods [35] . A LacZ reporter gene cassette, flanked by two FRT sequences, was introduced before the first exon of the Rcor2 gene locus, and first several exons were flanked by two LoxP sites in Rcor2 LacZ mice ( Supplementary Fig. 1a ). With these Rcor2 LacZ mice, we generated the wild-type Rcor2 flox/flox (Rcor2 fl/fl ) mice by Flippase splicing. After this, we were able to investigate conditional loss-of-function of Rcor2 (Rcor2 cko ) in specific tissues on Cre recombination in Rcor2 fl/fl mice ( Supplementary Fig. 1a ). First, by LacZ enzymatic activity assay, we examined the expression and localization of Rcor2 during embryonic development. X-gal staining of Rcor2 LacZ/+ embryos at embryonic day 11.5 (E11.5) revealed Rcor2 was mainly and highly expressed in the CNS, including the brain and spinal cord ( Fig. 1a ), indicating that Rcor2 may play an important role in the neural development of embryos. Western blot analysis of Rcor2 expression levels revealed decreased expression of Rcor2 in embryonic brains during development, suggesting Rcor2 may primarily function in early brain development ( Fig. 1b ). To examine the endogenous Rcor2 expression pattern during cortical development, we performed in situ hybridization and immunostaining by an RNA probe or antibody, and both were specific by no signals detected in the neural lineage-knockout Rcor2 fl/fl Nes Cre (Rcor2 cko ) cortex ( Supplementary Fig. 1b,c ). At early stages of brain development, Rcor2 messenger RNA and protein levels were high in mostly all cells in the wild-type mice cortex ( Fig. 1c,d ). Similar to the protein expression pattern as we observed in western blotting results ( Fig. 1b ), Rcor2 mRNA levels were also decreased as brains developed ( Fig. 1c ). As a transcriptional co-repressor, Rcor2 localized mainly in the cell nucleus, as expected ( Fig. 1d ). Interestingly, Rcor2 exhibited diverse subcellular localizations at different stages of the cell cycle, suggesting that it might directly play a role in cell division process. We observed Rcor2 protein puncta in the nucleus in interphase RG cells and localized mainly in chromosomes in metaphase RGCs in the ventricular zone (VZ). When cells entered anaphase, Rcor2 partially translocated to the space between two sets of separated chromosomes ( Fig. 1d ). Our observations are similar to the localization patterns of histone demethylase LSD1 in ESCs in previous studies, which showed LSD1 can regulate short timescale gene expressions during cell cycle progression by being recruited to or displaced from chromatin [36] , suggesting that Rcor2 may directly regulate NSC or NPC divisions by associating with LSD1. Taken together, Rcor2 is dominantly expressed in the CNS during mouse development and its expression pattern in the NSCs or NPCs exhibits regional differences in cell cycle, suggesting that Rcor2 may play an important role in regulating cerebral cortex development. 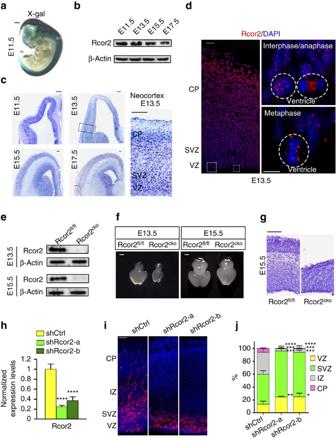Figure 1: Rcor2 expresses in the CNS and regulates cortical development. (a) X-gal staining to detect Rcor2 expression patterns. Whole-embryo staining at E11.5 stage shows Rcor2 is mainly expressed in the CNS. Scale bar, 1 mm. (b) Western blot analysis of Rcor2 expression levels during brain development. The decreased expression of Rcor2 with embryonic development is noteworthy. β-Actin is used as an endogenous control. (c)In situhybridization to detect endogenousRcor2mRNA expression patterns in cortical development at E11.5, E13.5, E15.5 and E17.5. Insets show high-magnification image of Rcor2 expression in the neocortex at E13.5. VZ, ventricular zone; SVZ, subventricular zone; CP, cortical plate. Scale bar, 100 μm. (d) Confocal images of immunofluorescence to detect cellular localization of Rcor2 in the neocortex at E13.5. Rcor2 localized mainly in the nucleus at interphase and metaphase, and localized between separated chromosomes in anaphase of dividing cells in VZ. Dotted lines circle the shape of nuclei. Scale bar, 5 μm. (e) Western blot analysis of Rcor2 expression level in Rcor2fl/fland Rcor2ckobrains at E13.5 and E15.5, respectively. Rcor2 expression was depleted in Rcor2ckobrains. β-Actin is used as an endogenous control. (f) Representative images of Rcor2fl/fland Rcor2ckobrain size at different stages of development. Rcor2ckomice show severe brain growth retardation at E13.5 and E15.5. Scale bar, 1 mm. (g) Representative images of Rcor2fl/fland Rcor2ckocortex at E15.5 by Nissl staining. Structural abnormalities of lamination with reduced cortical thickness are observed in Rcor2ckocortex. Scale bar, 200 μm. (h) RT–qPCR analysis of knockdown efficiencies of the two shRNAs targeting Rcor2. Transcripts were normalized to the control group. Data are shown as mean±s.e.m.,t-test, ****P<0.0001,n=3. (i) Confocal images of E16.5 cortical sections electroporated with shControl (red), shRcor2-a (red) and shRcor2-b (red) plasmids at E13.5. Knockdown of Rcor2 results in impaired cortical development. IZ, intermediate zone. Scale bar, 20 μm. (j) Quantification of the percentage of RFP+cells in different regions of the developing neocortex after electroporation as shown ini. proportion of RFP+cells in different zones (yaxis). Data are shown as mean±s.e.m.,t-test, *P<0.05, **P<0.01, ***P<0.001 and ****P<0.0001,n=3 individual experiments. Figure 1: Rcor2 expresses in the CNS and regulates cortical development. ( a ) X-gal staining to detect Rcor2 expression patterns. Whole-embryo staining at E11.5 stage shows Rcor2 is mainly expressed in the CNS. Scale bar, 1 mm. ( b ) Western blot analysis of Rcor2 expression levels during brain development. The decreased expression of Rcor2 with embryonic development is noteworthy. β-Actin is used as an endogenous control. ( c ) In situ hybridization to detect endogenous Rcor2 mRNA expression patterns in cortical development at E11.5, E13.5, E15.5 and E17.5. Insets show high-magnification image of Rcor2 expression in the neocortex at E13.5. VZ, ventricular zone; SVZ, subventricular zone; CP, cortical plate. Scale bar, 100 μm. ( d ) Confocal images of immunofluorescence to detect cellular localization of Rcor2 in the neocortex at E13.5. Rcor2 localized mainly in the nucleus at interphase and metaphase, and localized between separated chromosomes in anaphase of dividing cells in VZ. Dotted lines circle the shape of nuclei. Scale bar, 5 μm. ( e ) Western blot analysis of Rcor2 expression level in Rcor2 fl/fl and Rcor2 cko brains at E13.5 and E15.5, respectively. Rcor2 expression was depleted in Rcor2 cko brains. β-Actin is used as an endogenous control. ( f ) Representative images of Rcor2 fl/fl and Rcor2 cko brain size at different stages of development. Rcor2 cko mice show severe brain growth retardation at E13.5 and E15.5. Scale bar, 1 mm. ( g ) Representative images of Rcor2 fl/fl and Rcor2 cko cortex at E15.5 by Nissl staining. Structural abnormalities of lamination with reduced cortical thickness are observed in Rcor2 cko cortex. Scale bar, 200 μm. ( h ) RT–qPCR analysis of knockdown efficiencies of the two shRNAs targeting Rcor2. Transcripts were normalized to the control group. Data are shown as mean±s.e.m., t -test, **** P <0.0001, n =3. ( i ) Confocal images of E16.5 cortical sections electroporated with shControl (red), shRcor2-a (red) and shRcor2-b (red) plasmids at E13.5. Knockdown of Rcor2 results in impaired cortical development. IZ, intermediate zone. Scale bar, 20 μm. ( j ) Quantification of the percentage of RFP + cells in different regions of the developing neocortex after electroporation as shown in i . proportion of RFP + cells in different zones ( y axis). Data are shown as mean±s.e.m., t -test, * P <0.05, ** P <0.01, *** P <0.001 and **** P <0.0001, n =3 individual experiments. Full size image Rcor2 regulates neurogenesis during cortical development Next, we adopted Rcor2 cko mice to study Rcor2’s role by conditional loss-of-function in neural lineage ( Supplementary Fig. 1a ). Western blot analysis of brains at E13.5 and E15.5 confirmed the expression of Rcor2 is completely depleted in Rcor2 cko brains ( Fig. 1e ). Investigation of the Rcor2 cko embryos revealed that the brain sizes were greatly decreased compared with the control (Rcor2 fl/fl ) embryos at respective developmental stages ( Fig. 1f ). Representative Nissl staining of Rcor2 fl/fl and Rcor2 cko brains slices at different developmental stages exhibited not only significantly reduced thickness of the cortex but also structural abnormalities of layers on Rcor2 depletion ( Fig. 1g and Supplementary Fig. 1d,e ), suggesting that depletion of Rcor2 affects neocortical development. For further confirmation, in-utero electroporation of two red fluorescent protein (RFP)–short hairpin RNAs (shRNAs) targeting different sites of Rcor2 mRNA were performed at the lateral ventricle in brains at E13.5, respectively, both of which could efficiently reduce Rcor2 expression level by 70% compared with the control group ( Fig. 1h ). Disruption of Rcor2 resulted in significant accumulation of RFP + cells at the VZ and subventricular zone (SVZ) regions, whereas it resulted in a dramatic reduction at the intermediate zone and cortical plate regions at E16.5, indicating impaired cortical development on Rcor2 downregulation ( Fig. 1i,j ). Moreover, the cortical developmental defects caused by Rcor2 knockdown could be rescued by electroporation of Rcor2 overexpression plasmid, but not Rcor1 expression, the homologue of Rcor2, which plays important roles in pyramidal cortical neuron development as previously reported ( Supplementary Fig. 1f,g ) [30] . All the results above suggest that Rcor2 directly plays a critical role in regulating embryonic cortical development, which is distinguishable from Rcor1. Rcor2 regulates cortical NSC/NPC proliferation Given the profound effects of Rcor2 on cortical development, we examined the proliferation and neurogenesis capacities of NSCs/NPCs on Rcor2 depletion during cortical development. Compared with the control group, decreased expressions of NPC markers Sox2 and Nestin were observed by immunostaining in Rcor2 cko cortex at E13.5 ( Fig. 2a,b and Supplementary Fig. 2a ). In addition, the population of intermediate progenitor cells (IPCs) identified by Tbr2 staining was also reduced on Rcor2 depletion ( Fig. 2c,d ). Reverse transcriptase–quantitative PCR (RT–qPCR) analysis using the developing neocortex samples at E13.5 and E15.5 also exhibit similar results ( Supplementary Fig. 2b ). To further confirm the observations above, we checked the expressions of Nestin, Sox2 and Tbr2 in the in-vitro -cultured Rcor2 fl/fl and Rcor2 cko NPCs established from Rcor2 fl/fl and Rcor2 cko ESC lines by immunostaining, which were similar to our in vivo observations ( Fig. 2e ). Above all, both in-vivo and in-vitro results suggest that NPC and IPC populations are significantly affected on Rcor2 knockout, which may result in proliferation defects during cortical development. 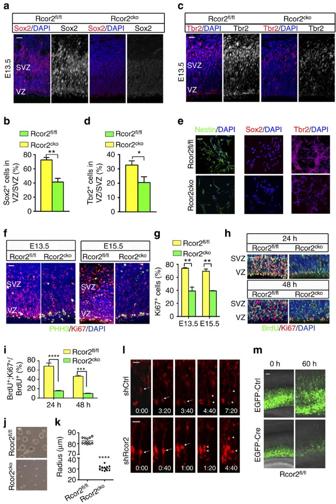Figure 2: Rcor2 regulates cortical NSC/NPC population and proliferation during development. (a) Immunostaining images of Sox2 at E13.5. Sox2 is dramatically reduced on Rcor2 depletion. VZ, ventricular zone; SVZ, subventricular zone. Scale bar, 20 μm. (b) Quantification of Sox2+cell ratios in VZ/SVZ regions shown ina. Data are shown as mean±s.e.m.,t-test, **P<0.01,n=3 individual experiments. (c) Confocal images of Tbr2 expression at E13.5. Tbr2 is dramatically reduced on Rcor2 depletion. Scale bar, 20 μm. (d) Quantification of Tbr2+cell ratios in VZ/SVZ regions shown inc, respectively. Data are shown as mean±s.e.m.,t-test, *P<0.05,n=3 individual experiments. (e) Immunostaining images of Nestin, Sox2 and Tbr2 in cultured Rcor2fl/fland Rcor2ckoNPCs, all of which exhibit significantly reduced expression in the Rcor2ckoNPCs. Scale bar, 20 μm. (f) Confocal images of immunofluorescence for Ki67 and PHH3 in Rcor2fl/fland Rcor2ckocortex at E13.5 and E15.5. Ki67 signals (red), but not PHH3 signals (green), are dramatically reduced in Rcor2ckodeveloping brains. Scale bar, 20 μm. (g) Quantification of Ki67+cells in the VZ/SVZ regions of the developing neocortex as shown inf. Data are shown as mean±s.e.m.,t-test, **P<0.01,n=3 separate stainings from three independent brains. (h) Confocal images of BrdU (green) and Ki67 (red) staining in Rcor2fl/fland Rcor2ckocortex 24 and 48 h after BrdU incorporation. Scale bar, 100 μm. (i) Quantification of the cell cycle exit by percentage of BrdU+and Ki67+NPCs divided by BrdU+cells shown inh. Data are shown as mean±s.e.m.,t-test, ***P<0.001 and ****P<0.0001,n=3 individual experiments. (j,k) Representative images (j) and quantification of (k) of Rcor2fl/fland Rcor2ckoneurosphere sizes. The neurospheres’radius of Rcor2ckoare much smaller than those of Rcor2fl/fl,t-test, ****P<0.0001,n=12. Scale bar, 50 μm. (l) Representative time-lapse imaging of the RGC dividing process in the sections of the cerebral cortex electroporated with RFP-shControl (upper panels) and RFP-shRcor2 (lower panels). The radial glial dividing pattern is abnormal on Rcor2 knockdown, resulting in cell death. Arrows, mother RGCs. Arrowheads, two daughter cells. Scale bar, 50 μm. (m) Representative time-lapse images of Rcor2fl/flcortex sections electroporated with EGFP-Control (upper panels) and EGFP-Cre (lower panels). Loss of cells is observed with Rcor2 knockout by Cre recombinase electroporation. Scale bar, 50 μm. Figure 2: Rcor2 regulates cortical NSC/NPC population and proliferation during development. ( a ) Immunostaining images of Sox2 at E13.5. Sox2 is dramatically reduced on Rcor2 depletion. VZ, ventricular zone; SVZ, subventricular zone. Scale bar, 20 μm. ( b ) Quantification of Sox2 + cell ratios in VZ/SVZ regions shown in a . Data are shown as mean±s.e.m., t -test, ** P <0.01, n =3 individual experiments. ( c ) Confocal images of Tbr2 expression at E13.5. Tbr2 is dramatically reduced on Rcor2 depletion. Scale bar, 20 μm. ( d ) Quantification of Tbr2 + cell ratios in VZ/SVZ regions shown in c , respectively. Data are shown as mean±s.e.m., t -test, * P <0.05, n =3 individual experiments. ( e ) Immunostaining images of Nestin, Sox2 and Tbr2 in cultured Rcor2 fl/fl and Rcor2 cko NPCs, all of which exhibit significantly reduced expression in the Rcor2 cko NPCs. Scale bar, 20 μm. ( f ) Confocal images of immunofluorescence for Ki67 and PHH3 in Rcor2 fl/fl and Rcor2 cko cortex at E13.5 and E15.5. Ki67 signals (red), but not PHH3 signals (green), are dramatically reduced in Rcor2 cko developing brains. Scale bar, 20 μm. ( g ) Quantification of Ki67 + cells in the VZ/SVZ regions of the developing neocortex as shown in f . Data are shown as mean±s.e.m., t -test, ** P <0.01, n =3 separate stainings from three independent brains. ( h ) Confocal images of BrdU (green) and Ki67 (red) staining in Rcor2 fl/fl and Rcor2 cko cortex 24 and 48 h after BrdU incorporation. Scale bar, 100 μm. ( i ) Quantification of the cell cycle exit by percentage of BrdU + and Ki67 + NPCs divided by BrdU + cells shown in h . Data are shown as mean±s.e.m., t -test, *** P <0.001 and **** P <0.0001, n =3 individual experiments. ( j , k ) Representative images ( j ) and quantification of ( k ) of Rcor2 fl/fl and Rcor2 cko neurosphere sizes. The neurospheres’radius of Rcor2 cko are much smaller than those of Rcor2 fl/fl , t -test, **** P <0.0001, n =12. Scale bar, 50 μm. ( l ) Representative time-lapse imaging of the RGC dividing process in the sections of the cerebral cortex electroporated with RFP-shControl (upper panels) and RFP-shRcor2 (lower panels). The radial glial dividing pattern is abnormal on Rcor2 knockdown, resulting in cell death. Arrows, mother RGCs. Arrowheads, two daughter cells. Scale bar, 50 μm. ( m ) Representative time-lapse images of Rcor2 fl/fl cortex sections electroporated with EGFP-Control (upper panels) and EGFP-Cre (lower panels). Loss of cells is observed with Rcor2 knockout by Cre recombinase electroporation. Scale bar, 50 μm. Full size image Next, we examined why NPC/IPC populations reduced on Rcor2 depletion. Immunostainings followed by quantification of cell proliferation markers Ki67 and phospho-histone H3 (PHH3) were performed in both Rcor2 fl/fl and Rcor2 cko developing cortex. Although PHH3 signals were not significantly affected, dramatically reduced Ki67 signals were observed in the VZ and SVZ regions on Rcor2 knockout during development ( Fig. 2f,g and Supplementary Fig. 2c left panel), indicating that depletion of Rcor2 would significantly affect proliferative cell numbers during cortical development. However, we observed that the mitotic index increased in VZ/SVZ regions in Rcor2 cko cortex ( Supplementary Fig 2c right panel), which is a result from decrease of Ki67 + cells compared with wild type, but no obvious changes of PHH3 + cell ( Fig. 2g and Supplementary Fig. 2c left panel). For further confirmation, we performed cell cycle exit analysis in Rcor2 fl/fl and Rcor2 cko brains at E13.5, respectively. Pulse-labelling cortex were analysed 24 or 48 h after 5-bromodeoxyuridine (BrdU) incorporation and Ki67 was used to identify cells that entered the following cell cycles ( Fig. 2h ). We found that 68.33±6.73% Rcor2 fl/fl NPCs and 15.28±1.02% Rcor2 cko NPCs in VZ/SVZ were able to undergo further rounds of cell division in the next 24 h. At 48 h after BrdU pulsing, only 9.71±0.84% Rcor2 cko NPCs were still in the cell cycles compared with 46.44±2.08% Rcor2 fl/fl NPCs ( Fig. 2i ), suggesting that cortical NPCs exit cell cycle at earlier time with Rcor2 depletion during development. In vitro , the neurosphere sizes of both Rcor2 fl/fl and Rcor2 cko NPCs were compared, which were significantly reduced on Rcor2 disruption ( Fig. 2j,k ). To examine the divisions of the cultured NPCs directly, we labelled the Rcor2 fl/fl and Rcor2 cko NPCs with green fluorescent protein (GFP)-expressing retrovirus (retro-GFP), which infected only dividing cells, and monitored the division process till 98 h after virus infection. To our observation, GFP + cells divided robustly in the wild-type group; however, the GFP + cells increased much more slowly on Rcor2 depletion ( Supplementary Fig. 2d,e ). We also performed cell cycle exit analysis by BrdU incorporation followed by Ki67 antibody staining in the cultured Rcor2 fl/fl and Rcor2 cko NPCs, respectively, which also showed earlier cell cycle exit on Rcor2 depletion ( Supplementary Fig. 2f,g ). To further dissect Rcor2’s role in NPC proliferation regulation, time-lapse imaging of the RGC dividing process was recorded after Rcor2 knockdown by specific shRNAs mentioned above ( Fig. 1h ). RGCs with Rcor2 knockdown showed interkinetic nuclear migration defect and the daughter cells showed apoptosis after separation ( Fig. 2l ), suggesting that Rcor2 is required for radial glia maintenance and cell division. In addition, we also knocked out Rcor2 by electroperating EGFP-Cre and EGFP-Control plasmids in Rcor2 fl/fl mouse embryos at E13.5 and recorded NPC proliferation in neocortex sections for 60 h, respectively. Compared with the control group in which robust cell proliferation and migration were observed, Rcor2 knockout NPC/IPCs generated fewer daughter cells ( Fig. 2m ). Immunostaining results showed enhanced Caspase 3 signals among Rcor2 cko neocortex compared with Rcor2 fl/fl cortex at E15.5 ( Supplementary Fig. 2h ). Significantly increased cell death was also observed in both cultured NPCs and neurons on Rcor2 knockout by TdT-mediated dUTP nick end labelling assays ( Supplementary Fig. 2i and 2j ). All together, these results suggest that Rcor2 plays an important role in cortical development via regulating NSC/NPC proliferation and maintenance. Rcor2 regulates cortical neurogenesis during development Given the observation of reduced NPC proliferation on Rcor2 depletion, we checked the expressions of neuronal markers in Rcor2 fl/fl and Rcor2 cko cortex at E15.5. On Rcor2 depletion, a consistent reduction in both Dcx + /Satb2 + /Tbr1 + cell numbers and Dcx + /Satb2 + /Tbr1 + -containing layer thickness was observed during cortical development ( Fig. 3a and Supplementary Fig. 3a ). Quantification confirmed dramatic decreases of Satb2 + and Tbr1 + cells, which are postmitotic pyramidal neurons, in Rcor2 cko developing neocortex compared with Rcor2 fl/fl ( Fig. 3b ). Western blot analysis also confirmed downregulation of the neuronal markers mentioned above ( Fig. 3c ), indicating reduction of NPC pool caused by Rcor2 depletion leads to reduced cortical neurons during development. In addition, we also assessed the fate of cells with Rcor2 downregulation by in-utero electroporation assay. Three days after injection of RFP–shRNAs targeting Rcor2 mRNA, we found that most RFP + cells localized in VZ/SVZ ( Fig. 1i,j ) and some of these cells were Pax6 + cells ( Supplementary Fig. 3b ). However, the ratio of Pax6 + cells among Rcor2-knockdown cells was greatly reduced compared with control samples ( Supplementary Fig. 3c ), which was consistent with the results that Rcor2 depletion reduced the NPC pool in mouse developing cortex ( Fig. 2a,b ). Immunostained with newborn neuron marker Dcx, we found that some of the RFP + cells were Dcx + ( Supplementary 3d ) and the ratio of Dcx + cells among RFP + cells was also significantly decreased ( Supplementary 3e ), indicating that Rcor2 depletion impaired neurogenesis, which is consistent with the observation in Rcor2 cko mice ( Fig. 3 ). 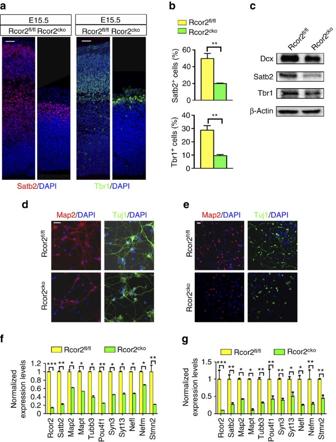Figure 3: Rcor2 regulates cortical neurogenesis during development. (a) Confocal images of Satb2 and Tbr1 expressions in Rcor2fl/fland Rcor2ckocortex at E15.5, which exhibit significant reduction on Rcor2 knockout. Scale bar, 50 μm. (b) Quantification of Satb2+and Tbr1+cells in Rcor2fl/fland Rcor2ckocortex at E15.5 inaindicates Satb2 and Tbr1 expressions are decreased on Rcor2 depletion during development. Data are shown as mean±s.e.m.,t-test, **P<0.01,n=3 individual experiments. (c) Western blot to analyse Dcx, Satb2 and Tbr1 expressions in Rcor2fl/fland Rcor2ckocortex at E15.5. β-Actin is used as an endogenous control. (d) Representative images of Map2 and Tuj1 immunostaining in cultured neurons directly dissociated from Rcor2fl/fland Rcor2ckobrain cortex at E15.5. Decreased expression of both markers and reduced neurofilaments can be observed in Rcor2ckocultured neurons. Scale bar, 20 μm. (e) Confocal images ofin-vitrocultured Rcor2fl/fland Rcor2ckoNPCs 5 days post spontaneous differentiation using neuronal marker Map2 and Tuj1 antibodies, both of which are significantly reduced in the differentiated Rcor2ckoNPCs. Scale bar, 20 μm. (f,g) RT–qPCR analysis of neuronal markers expression in both Rcor2fl/fland Rcor2ckoneocortex at E15.5 stage (f) andin-vitro-cultured Rcor2fl/fland Rcor2ckoNPCs 5 days post spontaneous differentiation (g). Transcripts were normalized to Rcor2fl/flgroup. Data are shown as mean±s.d.,t-test, *P<0.05, **P<0.01 and ***P<0.001,n=3. Figure 3: Rcor2 regulates cortical neurogenesis during development. ( a ) Confocal images of Satb2 and Tbr1 expressions in Rcor2 fl/fl and Rcor2 cko cortex at E15.5, which exhibit significant reduction on Rcor2 knockout. Scale bar, 50 μm. ( b ) Quantification of Satb2 + and Tbr1 + cells in Rcor2 fl/fl and Rcor2 cko cortex at E15.5 in a indicates Satb2 and Tbr1 expressions are decreased on Rcor2 depletion during development. Data are shown as mean±s.e.m., t -test, ** P <0.01, n =3 individual experiments. ( c ) Western blot to analyse Dcx, Satb2 and Tbr1 expressions in Rcor2 fl/fl and Rcor2 cko cortex at E15.5. β-Actin is used as an endogenous control. ( d ) Representative images of Map2 and Tuj1 immunostaining in cultured neurons directly dissociated from Rcor2 fl/fl and Rcor2 cko brain cortex at E15.5. Decreased expression of both markers and reduced neurofilaments can be observed in Rcor2 cko cultured neurons. Scale bar, 20 μm. ( e ) Confocal images of in-vitro cultured Rcor2 fl/fl and Rcor2 cko NPCs 5 days post spontaneous differentiation using neuronal marker Map2 and Tuj1 antibodies, both of which are significantly reduced in the differentiated Rcor2 cko NPCs. Scale bar, 20 μm. ( f , g ) RT–qPCR analysis of neuronal markers expression in both Rcor2 fl/fl and Rcor2 cko neocortex at E15.5 stage ( f ) and in-vitro -cultured Rcor2 fl/fl and Rcor2 cko NPCs 5 days post spontaneous differentiation ( g ). Transcripts were normalized to Rcor2 fl/fl group. Data are shown as mean±s.d., t -test, * P <0.05, ** P <0.01 and *** P <0.001, n =3. Full size image Immunostaining of Map2 and Tuj1 were also performed in the primary cultured neurons dissociated from Rcor2 fl/fl and Rcor2 cko cortex at E15.5, which showed greatly decreased expression of both markers and significantly reduced neurofilaments on Rcor2 depletion ( Fig. 3d ). Similar results were also found in the in-vitro -cultured Rcor2 cko NPCs subjected to differentiation for 5 days ( Fig. 3e ). Moreover, RT–qPCR analysis of in vivo and in vitro samples also exhibited significant downregulation of neuronal markers such as Map2 , Tubb3 and Pou4f1 ( Fig. 3f,g ). Thus, our data suggest that Rcor2 mediates neurogenesis both in vivo and in vitro ; hence, depletion of Rcor2 leads to affected proliferation of NPC and production of neurons during development. Rcor2 regulates neurogenesis as a co-repressor of LSD1 Previous studies indicate that Rcor2 works as a co-repressor, closely related to LSD1 complex, to facilitate its nucleosomal demethylase activity [34] . Given the significantly reduced neurogenesis on Rcor2 disruption, we constructed Rcor2 Flag knock-in mice in which 3 × Flag sequences were introduced behind the start codon of Rcor2 protein by CRISPR/Cas9 system, to identify the targets of Rcor2 during cortical development ( Fig. 4a ). Western blot analysis confirmed FLAG expression in Rcor2 Flag knock-in brains and stable expression of endogenous Rcor2 with a Flag tag ( Fig. 4b ). Immunostaining of Flag, Rcor2 and Lsd1 antibodies in Rcor2 Flag cortex at E11.5 also confirmed Flag antibody co-immunostained with Rcor2 antibody and LSD1 in all cells of the neocortex ( Supplementary Fig. 4a ) and the protein localization was similar to the staining results using Rcor2 antibody ( Fig. 1d ). Immunoprecipitation (IP) followed by western blot analysis revealed that Rcor2-Flag and LSD1 could interact with each other in Rcor2 Flag brains ( Supplementary Fig. 4b ), which may function in a large complex containing multiple components as previous studies [37] , [38] . All results above suggest the expression of Flag in Rcor2 Flag mice could indicate the endogenous expression of Rcor2, which serves as a co-repressor of LSD1 complex in the mouse embryonic brains. 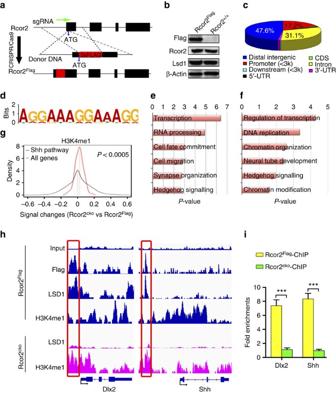Figure 4: ChIP-seq analysis of Rcor2 enrichments in genome-wide scale reveals direct binding of Rcor2 at regulatory regions of genes related to Shh signalling pathway. (a) Schematic overview of strategy to generate an Rcor2Flagknock-in allele by CRISPR/Cas9. The sgRNA sequence site is shown as a green arrowhead. The start codon of Rcor2 is indicated and capitalized. The oligo donor contained 50 bp homologies on both sides flanking the DSB, in which 3 × Flag sequences are labelled as a red box. (b) Western blot analysis to validate FLAG, RCOR2 and LSD1 expressions in Rcor2Flagknock-in neocortex using Flag-M2 antibody. β-Actin was used as an endogenous control. (c) Pie chart depicts distribution of Rcor2 occupancies in genome-wide scale in FLAG ChIP-seq results using Rcor2Flagknock-in neocortex at E13.5. (d) WebLogos of consensus binding motifs of Rcor2 generated by Multiple EM for Motif Elicitation (MEME) motif analysis tool. (e) GO analysis for Rcor2-binding regions in genome-wide scale revealed by Flag ChIP-seq results using Rcor2Flagbrain. (f) GO analysis for LSD1 occupancy in genome-wide scale revealed by LSD1 ChIP-seq results using Rcor2Flagbrain. (g) Density plots analysis of H3K4me1 signal change in promoter regions (−2- to∼0.5 kb from TSS) on Rcor2 depletion. Compared with all genes, the change of H3K4me1 signal is significantly (P<0.0005, Kolmogorov–Smirnov test) enhanced in the promoter regions of Shh pathway-related genes on Rcor2 depletion. H3K4me1 signal change on Rcor2 depletion (xaxis); H3K4me1 signal density (yaxis). (h) Gene tracks of Rcor2, LSD1 and H3K4me1 enrichments by ChIP-seq analysis at core promoter regions of Dlx2 and upstream regulatory regions of Shh, which are closely related to Shh signalling. (i) ChIP–qPCR analysis of Rcor2Flagand Rcor2ckocortex at E13.5 using specific FLAG-M2 antibody. Significant enrichments of the Rcor2 at the regulatory regions of Dlx2 and Shh gene locus detected ingin the Rcor2flagsamples are worth noting. Fold enrichments of Rcor2 occupancy compared with input (yaxis). Data are shown as mean±s.d.,t-test, ***P<0.001,n=3. Figure 4: ChIP-seq analysis of Rcor2 enrichments in genome-wide scale reveals direct binding of Rcor2 at regulatory regions of genes related to Shh signalling pathway. ( a ) Schematic overview of strategy to generate an Rcor2 Flag knock-in allele by CRISPR/Cas9. The sgRNA sequence site is shown as a green arrowhead. The start codon of Rcor2 is indicated and capitalized. The oligo donor contained 50 bp homologies on both sides flanking the DSB, in which 3 × Flag sequences are labelled as a red box. ( b ) Western blot analysis to validate FLAG, RCOR2 and LSD1 expressions in Rcor2 Flag knock-in neocortex using Flag-M2 antibody. β-Actin was used as an endogenous control. ( c ) Pie chart depicts distribution of Rcor2 occupancies in genome-wide scale in FLAG ChIP-seq results using Rcor2 Flag knock-in neocortex at E13.5. ( d ) WebLogos of consensus binding motifs of Rcor2 generated by Multiple EM for Motif Elicitation (MEME) motif analysis tool. ( e ) GO analysis for Rcor2-binding regions in genome-wide scale revealed by Flag ChIP-seq results using Rcor2 Flag brain. ( f ) GO analysis for LSD1 occupancy in genome-wide scale revealed by LSD1 ChIP-seq results using Rcor2 Flag brain. ( g ) Density plots analysis of H3K4me1 signal change in promoter regions (−2- to ∼ 0.5 kb from TSS) on Rcor2 depletion. Compared with all genes, the change of H3K4me1 signal is significantly ( P <0.0005, Kolmogorov–Smirnov test) enhanced in the promoter regions of Shh pathway-related genes on Rcor2 depletion. H3K4me1 signal change on Rcor2 depletion ( x axis); H3K4me1 signal density ( y axis). ( h ) Gene tracks of Rcor2, LSD1 and H3K4me1 enrichments by ChIP-seq analysis at core promoter regions of Dlx2 and upstream regulatory regions of Shh, which are closely related to Shh signalling. ( i ) ChIP–qPCR analysis of Rcor2 Flag and Rcor2 cko cortex at E13.5 using specific FLAG-M2 antibody. Significant enrichments of the Rcor2 at the regulatory regions of Dlx2 and Shh gene locus detected in g in the Rcor2 flag samples are worth noting. Fold enrichments of Rcor2 occupancy compared with input ( y axis). Data are shown as mean±s.d., t -test, *** P <0.001, n =3. Full size image Using the Flag M2 antibody, we micro-dissected Rcor2 Flag brains at E13.5 to isolate neocortex followed by chromatin IP sequencing (ChIP-seq) analysis ( Supplementary Fig. 4c ) and identified 1,994 Rcor2-binding peaks in genome-wide scale. Further analysis showed Rcor2-binding sites are mostly (47.6%) enriched in distal intergenic regions, followed by introns and promoters, the ratios of which are 31.1% and 17.2% respectively ( Fig. 4c ). Binding motif analysis by Multiple EM for Motif Elicitation demonstrates enrichments of AG-rich motifs of Rcor2-binding regions ( Fig. 4d ). Gene Ontology (GO) analysis of Rcor2 occupancy regions showed significant ( P <0.01) enrichment of terms related to transcription, cell fate commitment, cell migration and synaptic organization ( Fig. 4e ), suggesting Rcor2 may directly regulate the transcriptional activity of specific genes involved in neurogenesis during cortical development. In addition, significant ( P <0.01) enrichment of terms related to Hedgehog signalling could also be observed in GO analysis of Rcor2 occupancy ( Fig. 4e ), indicating Rcor2 may primarily target genes related to Shh signalling pathway. We also performed ChIP-seq analysis in the dissected Rcor2 Flag neocortex at E13.5 using LSD1 antibody. Besides terms related to regulation of transcription, chromatin organization and neural tube development, GO analysis of LSD1 targets also revealed significant ( P <0.01) enrichment of Hedgehog signalling ( Fig. 4f ). Moreover, we could observe enhanced H3K4me1 signal in most regulatory regions of Shh pathway-related genes compared with all genes on Rcor2 knockout by H3K4me1 ChIP-seq analysis ( Fig. 4g ), further suggesting that Rcor2 and LSD1 form a complex, playing roles in Shh signalling pathway regulation. Detailed investigation of the binding profiles revealed that Rcor2 and LSD1 co-occupied the core promoter regions of Dlx2 and the upstream regulatory regions of Shh ( Fig. 4h ), as well as the promoters of Dlx5 and Ascl1 ( Supplementary Fig. 4d ), all of which are important for Shh signalling pathway. Coupled with H3K4me1 ChIP-seq results, we found that the regulatory regions of the above genes occupied by Rcor2 and LSD1 were with significantly reduced or even absent H3K4me1 enrichments in Rcor2 Flag neocortex ( Fig. 4h and Supplementary Fig. 4d ). On depletion of Rcor2, although LSD1 enrichments were dramatically decreased, these regions mentioned above exhibited significantly increased H3K4me1 signals ( Fig. 4h and Supplementary Fig. 4d ), suggesting that Rcor2 may directly target the upstream regulatory regions and recruit LSD1 complex to executive demethylation on H3K4 sites of these genes. ChIP–qPCR analysis further validated the ChIP-seq results above, which showed significant ( P <0.001) enrichments of Rcor2 in the core promoter regions or enhancers of genes mentioned above in Rcor2 Flag neocortex at E13.5 ( Fig. 4i and Supplementary Fig. 4e ). We also tested whether Rcor1 could functionally substitute for Rcor2 to repress the target genes. ChIP–qPCR analysis using Rcor1 antibody showed no significant enrichments of Rcor1 on Shh signalling-related genes ( Supplementary Fig. 4f ), further suggesting that Rcor1 may target distinct genes from Rcor2 to regulate cortical development. Taken together, our ChIP-seq results of Rcor2 Flag and Rcor2 cko neocortex demonstrate that Rcor2 working as a co-repressor of LSD1 complex could regulate the transcriptional activities of genes involved in neurogenesis and, more importantly, directly target genes important for Shh signalling pathway, such as Dlx2 and Shh . Shh pathway is highly activated in Rcor2-depleted cortex Next, to categorize gene expression changes due to the dysfunction of Rcor2, we performed RNA-sequencing (RNA-seq) to analyse the genome-wide changes on Rcor2 depletion at E13.5 and E15.5, respectively, in developing cortex ( Supplementary Fig. 4c ). Expression profile of Rcor2 showed RNA peaks of exons between the two LoxP sites were totally absent in Rcor2 cko cortex at E13.5 and E15.5, indicating successful excision of exons by Cre recombinase ( Supplementary Fig. 5a ). By comparing gene expression levels in wild-type and knockout samples at the same developmental stage, depletion of Rcor2 predominantly resulted in upregulation of genes, which further confirms its function as a transcriptional co-repressor ( Fig. 5a,b ). Importantly, we found significant upregulation of Dlx2 , Shh , Ptch1 , Gli1 , Nkx2.1 , Gsx2 and Ascl1 at E13.5 ( Fig. 5b ) and activation of Dlx2 , Shh, Nkx2.1 and Gsx2 at E15.5 ( Fig. 5c ) when Rcor2 was knocked out, suggesting that Shh signalling pathway is upregulated in both E13.5 and E15.5 samples due to the lack of Rcor2. In addition, genes involved in cortical neurogenesis, such as Emx1 , Tbr2 , Trnp1 , Foxg1 and Reln ( Fig. 5a,b ), were significantly downregulated on Rcor2 depletion, further suggesting Rcor2’s function in cortical neurogenesis regulation. 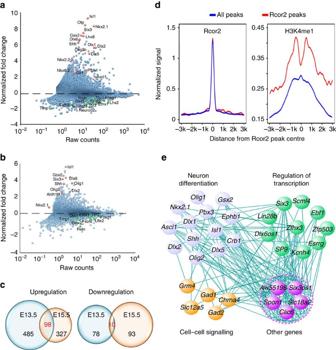Figure 5: Genome-wide expression changes on Rcor2 depletion in mouse developing cortex by RNA-seq analysis. (a,b) Scatter plot analysis of genome-wide expression profiles of Rcor2ckoversus Rcor2fl/flsamples at E13.5 (a) and E15.5 (b). Dots above or below the dash line indicate upregulated or downregulated genes on Rcor2 depletion, respectively. Red dots or green dots highlight the significantly differentially expressed genes on Rcor2 depletion. Raw counts (xaxis); gene expression fold changes on Rcor2 depletion (yaxis). (c) Venn diagrams of upregulated genes (left) and downregulated genes (right) in Rcor2ckosamples compared with Rcor2fl/flsamples. (d) The profiles of Rcor2 and H3k4me1 enrichments analysed in ChIP-seq results shown inFig. 3in regulatory regions of genome-wide scale (red) and of the upregulated genes (purple) according to RNA-seq results. (e) Correlation network of overlapped upregulated genes in both E13.5 and E15.5 samples. Lines indicate the correlations between two connected genes withR>0.55. Genes were analysed by GO analysis and divided into different categories. Figure 5: Genome-wide expression changes on Rcor2 depletion in mouse developing cortex by RNA-seq analysis. ( a , b ) Scatter plot analysis of genome-wide expression profiles of Rcor2 cko versus Rcor2 fl/fl samples at E13.5 ( a ) and E15.5 ( b ). Dots above or below the dash line indicate upregulated or downregulated genes on Rcor2 depletion, respectively. Red dots or green dots highlight the significantly differentially expressed genes on Rcor2 depletion. Raw counts ( x axis); gene expression fold changes on Rcor2 depletion ( y axis). ( c ) Venn diagrams of upregulated genes (left) and downregulated genes (right) in Rcor2 cko samples compared with Rcor2 fl/fl samples. ( d ) The profiles of Rcor2 and H3k4me1 enrichments analysed in ChIP-seq results shown in Fig. 3 in regulatory regions of genome-wide scale (red) and of the upregulated genes (purple) according to RNA-seq results. ( e ) Correlation network of overlapped upregulated genes in both E13.5 and E15.5 samples. Lines indicate the correlations between two connected genes with R >0.55. Genes were analysed by GO analysis and divided into different categories. Full size image In the RNA-seq results, 563 genes (485 upregulated and 78 downregulated) at E13.5 and 420 genes (327 upregulated and 93 downregulated) at E15.5 were differentially expressed on Rcor2 depletion as compared with the control samples ( P <0.01, fold changes >1.5; Fig. 5d ). GO term analysis of downregulated genes in E13.5 samples showed a significant ( P <0.01) enrichment of terms related to neuron differentiation (for example, neuron differentiation, neuron projection development, morphogenesis involved in neuron differentiation, axonogenesis and forebrain development) in the 78 downregulated genes ( Supplementary Fig. 5b ), similar to the enrichment of terms in E15.5 samples ( Supplementary Fig. 5c ). Notably, genes involved in chromatin assembly or nucleosome organization were significantly downregulated on Rcor2 depletion at E15.5 stage ( Supplementary Fig. 5c ), indicating Rcor2 may regulate gene activity involved in neurogenesis by affecting chromatin structure. Coupled with the aforementioned ChIP-seq results ( Fig. 4 ), we compared both Rcor2-Flag and H3K4me1 enrichment profiles in the regulatory regions of the upregulated genes shown in RNA-seq results with those of genome-wide scale. As the enrichments of Rcor2-Flag in the regulatory regions of upregulated genes could coincide well with those of genome-wide scale, the enrichments of H3K4me1 distributed near the regions of Rcor2 occupancy (however, absent from the Rcor2 peaks in the regulatory regions of genes; Fig. 5d ), further suggesting that Rcor2 directly regulate these genes’ activities by recruiting LSD1 complex, which would tolerate no methyl modifications on H3K4 sites. Among the 98 overlapping upregulated genes ( Fig. 5c ), expression correlation analysis exhibited that 68 gene expressions were positively correlated with other genes with a cutoff R -value (correlation coefficient) as 0.55, in which 13 genes were highly related to neuron differentiation, 10 genes were involved in transcription regulation and 5 genes were categorized to cell–cell signalling ( Fig. 5e and Supplementary Table S1 ), indicating that Rcor2 might regulate transcription, neuron differentiation and fate specification. Taken together, both ChIP-seq and RNA-seq results strongly demonstrate that Rcor2 could directly target genes involved in Shh signalling pathway, such as Shh and Dlx2 , to repress their transcriptional activities during cortical neurogenesis. Given the direct enrichments of Rcor2 on molecules involved in Shh signalling ( Figs 4 and 5 ), we validated the expression of genes involved in Shh signalling pathways on Rcor2 depletion. RT–qPCR analysis of both in-vivo neocortical samples and in-vitro -cultured NPCs revealed significant activation of Shh signalling pathway on Rcor2 depletion ( Fig. 6a and Supplementary Fig. 6a ). Immunostaining results showed the signals of Shh and its receptor Ptch1, which maintained low levels in Rcor2 fl/fl cortex during development as reported [19] , were both significantly enhanced with localization on the membrane of cortical cells on Rcor2 depletion ( Fig. 6b ). Strikingly, we found enrichment of Dlx2 signals at E15.5 in the neocortex on Rcor2 depletion ( Fig. 6c ), consistent with ChIP-seq and RNA-seq data. The staining observations above were validated by immunostaining in cultured Rcor2 cko NPCs in vitro , which also exhibited significantly enhanced expression of Shh, Ptch1 and Dlx2 ( Fig. 6d ). In addition, western blot analysis also confirmed the upregulation of the above genes related to Shh signalling on Rcor2 knockout during cortical development ( Fig. 6e ). Taken together, both in vivo and in vitro data above strongly suggest that Rcor2 plays an important role in repression of Shh signalling pathway. 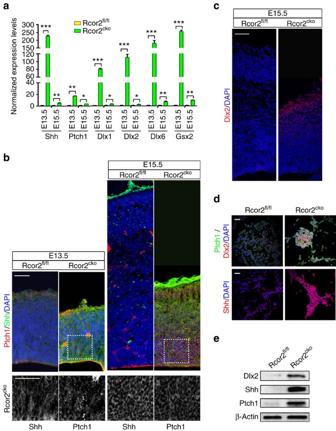Figure 6: Rcor2 regulates Shh signalling pathway during cortical development. (a) qPCR analysis of the expression of genes related to the Shh signalling pathway in the cortex of Rcor2fl/fland Rcor2ckobrains during development. Significant upregulation of these genes on Rcor2 depletion is noteworthy. Transcripts were normalized to Rcor2fl/flgroup. Data are shown as mean±s.d.,t-test, *P<0.05, **P<0.01 and ***P<0.001,n=3. (b) Confocal images of Shh and Ptch1 expressions in Rcor2fl/fland Rcor2ckocortex. Enhanced Shh and Ptch1 signals are observed in Rcor2ckocompared with Rcor2fl/flneocortex at E13.5 and E15.5. Insets show high-magnification images of the outlined regions. Scale bars, 50 μm. (c) Dlx2 expression in Rcor2fl/fland Rcor2ckocortex detected by immunofluorescence analysis at E15.5. Dlx2+cells were observed in the neocortex on Rcor2 depletion. Scale bars, 50 μm. (d) Confocal images of Shh, Ptch1 and Dlx2 expressions inin-vitro-cultured Rcor2ckoNPCs. Scale bar, 20 μm. (e) Western blot analysis of expression levels of Dlx2, Shh and Ptch1 in Rcor2fl/fland Rcor2ckocortex at E15.5. β-Actin is used as an endogenous control. Figure 6: Rcor2 regulates Shh signalling pathway during cortical development. ( a ) qPCR analysis of the expression of genes related to the Shh signalling pathway in the cortex of Rcor2 fl/fl and Rcor2 cko brains during development. Significant upregulation of these genes on Rcor2 depletion is noteworthy. Transcripts were normalized to Rcor2 fl/fl group. Data are shown as mean±s.d., t -test, * P <0.05, ** P <0.01 and *** P <0.001, n =3. ( b ) Confocal images of Shh and Ptch1 expressions in Rcor2 fl/fl and Rcor2 cko cortex. Enhanced Shh and Ptch1 signals are observed in Rcor2 cko compared with Rcor2 fl/fl neocortex at E13.5 and E15.5. Insets show high-magnification images of the outlined regions. Scale bars, 50 μm. ( c ) Dlx2 expression in Rcor2 fl/fl and Rcor2 cko cortex detected by immunofluorescence analysis at E15.5. Dlx2 + cells were observed in the neocortex on Rcor2 depletion. Scale bars, 50 μm. ( d ) Confocal images of Shh, Ptch1 and Dlx2 expressions in in-vitro -cultured Rcor2 cko NPCs. Scale bar, 20 μm. ( e ) Western blot analysis of expression levels of Dlx2, Shh and Ptch1 in Rcor2 fl/fl and Rcor2 cko cortex at E15.5. β-Actin is used as an endogenous control. Full size image Previous studies demonstrated that Shh, as a classic morphogen, plays important roles in dorsal–ventral specification during CNS development [19] , [39] . Next, we checked whether abnormally activated Shh signalling caused by Rcor2 depletion affected dorsal–ventral gene expression pattern during cortical development. Similar to our RNA-seq results ( Fig. 5b ), quantitative expression analysis also showed significant downregulation of dorsal marker genes such as Emx1 and Emx2 , and dramatically upregulated ventral marker genes including Nkx2.1 , Dlx6 , Olig2 and so on in E15.5 neocortex on Rcor2 depletion ( Supplementary Fig. 6b ). Besides the defects in excitatory neuron production on Rcor2 knockout during cortical development ( Fig. 3 and Supplementary Fig. 3a ), we also observed enriched expressions of interneuron markers, Calretinin and Somatostatin, in Rcor2 cko dorsal cortex at E15.5 by immunostaining ( Supplementary Fig. 6c ). These results strongly suggest that Rcor2 function in repression of Shh signalling pathway, thereby specifying dorsal–ventral gene expression patterns during cortical development, resulting in ectopic generation of cells that might be inhibitory neurons. Although using Nestin-driven conditional knockout mice is a typical choice for the central nerve system research, however, to further study Rcor2 function in neocortical development we generated Rcor2 fl/fl Emx1 Cre (Rcor2 Emx ) mice to specifically knock out Rcor2 in the neocortex [40] . We observed similar phenotype in Rcor2 Emx developing neocortex ( Supplementary Fig. 7 ), excluding the possibility that our observations in Rcor2 cko neocortex is caused by the side effects of Nestin-driven Rcor2 depletion and further confirming Rcor2’s important roles during neocortical development. Inhibition of Shh partially rescues Rcor2-depletion defects Given the profound fact that Rcor2 regulates cortical neurogenesis by repressing Shh and its downstream factor Dlx2 during development, we next asked whether inhibition of Shh could rescue the phenotypes caused by Rcor2 disruption. To test this, both specific shRNAs and inhibitor Cyclopamine [41] were adopted to inhibit Shh activity in the cortex electroporated with Rcor2 RFP–shRNAs. Electroporation of Shh shRNAs into the shRcor2 neocortex could partially rescue the neurogenesis defects caused by Rcor2 knockdown ( Fig. 7a,b ). Similarly, Cyclopamine treatment of the shRcor2 neocortex could also relieve such defects ( Fig. 7c,d ), suggesting that Rcor2 regulates cortical neurogenesis through regulating Shh signalling pathway. 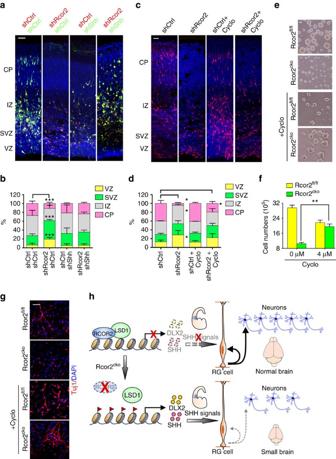Figure 7: Rcor2 regulates cortical development by inhibition of Shh. (a) Knockdown of Rcor2 impairs cortical neurogenesis, which can be partially rescued by knockdown of Shh during cortical development.In-uteroelectroporation with RFP-shControl (red)/GFP-shControl (green), RFP-shRcor2 (red)/GFP-shControl (green), RFP-shControl (red)/GFP-shShh (green) or RFP-shRcor2 (red)/GFP-shShh (green) plasmids was performed at E13.5. Cerebral sections were fixed and imaged at E16.5. VZ, ventricular zone; SVZ, subventricular zone; CP, cortical plate. Scale bar, 50 μm. (b) Quantification of the percentage of RFP+/GFP+cells in different regions of the developing cortex after electroporation shown ina. Data are shown as mean±s.e.m.,t-test, **P<0.01 and ***P<0.001,n=3 individual experiments. (c) Inhibition of Shh by Cyclopamine can partially rescue neurogenesis defects caused by Rcor2 downregulation during cortical development. Rcor2 was knocked down at the lateral ventricle in the brain byin-uteroelectroporation with RFP-shRcor2 plasmids at E13.5. Cerebral sections were collected at E14.5 and then treated with cyclopamine to inhibit Shh activity for 48 h. Scale bar, 50 μm. (d) Quantification of the percentage of RFP+cells in different regions of the developing neocortex after knockdown of Rcor2 or inhibition of Shh shown inc. Data are shown as mean±s.e.m.,t-test, *P<0.05,n=3 individual experiments. (e) Representative images depicting neurosphere size is partially rescued in thein-vitro-cultured Rcor2ckoNPCs after treatment with Cyclopamine. Scale bar, 50 μm. (f) Histogram depicting cell numbers ofin-vitro-cultured Rcor2fl/fland Rcor2ckoNPCs with or without Cyclopamine treatment for 48 h. Cells (5 × 105) are seeded initially. Data are shown as mean±s.e.m.,t-test, **P<0.01,n=3. (g) Confocal images of Tuj1 expression in the differentiated cells fromin-vitro-cultured Rcor2fl/fland Rcor2ckoNPCs with or without Cyclopamine treatment. Tuj1 expressions are partially restored in Cyclopamine-treated Rcor2ckocells. Scale bar, 20 μm. (h) Model of Rcor2 function in neurogenesis in the developing neocortex. Rcor2 safeguards cortical neurogenesis by recruiting LSD1 complex to the regulatory regions of Dlx2 and Shh genes, to inhibit the Shh pathway activation during development. The absence of Rcor2 leads to inhibition release of these genes and thus ectopic activation of Shh signalling in the developing neocortex, resulting in cortical neurogenesis defects. Figure 7: Rcor2 regulates cortical development by inhibition of Shh. ( a ) Knockdown of Rcor2 impairs cortical neurogenesis, which can be partially rescued by knockdown of Shh during cortical development. In-utero electroporation with RFP-shControl (red)/GFP-shControl (green), RFP-shRcor2 (red)/GFP-shControl (green), RFP-shControl (red)/GFP-shShh (green) or RFP-shRcor2 (red)/GFP-shShh (green) plasmids was performed at E13.5. Cerebral sections were fixed and imaged at E16.5. VZ, ventricular zone; SVZ, subventricular zone; CP, cortical plate. Scale bar, 50 μm. ( b ) Quantification of the percentage of RFP + /GFP + cells in different regions of the developing cortex after electroporation shown in a . Data are shown as mean±s.e.m., t -test, ** P <0.01 and *** P <0.001, n =3 individual experiments. ( c ) Inhibition of Shh by Cyclopamine can partially rescue neurogenesis defects caused by Rcor2 downregulation during cortical development. Rcor2 was knocked down at the lateral ventricle in the brain by in-utero electroporation with RFP-shRcor2 plasmids at E13.5. Cerebral sections were collected at E14.5 and then treated with cyclopamine to inhibit Shh activity for 48 h. Scale bar, 50 μm. ( d ) Quantification of the percentage of RFP + cells in different regions of the developing neocortex after knockdown of Rcor2 or inhibition of Shh shown in c . Data are shown as mean±s.e.m., t -test, * P <0.05, n =3 individual experiments. ( e ) Representative images depicting neurosphere size is partially rescued in the in-vitro -cultured Rcor2 cko NPCs after treatment with Cyclopamine. Scale bar, 50 μm. ( f ) Histogram depicting cell numbers of in-vitro -cultured Rcor2 fl/fl and Rcor2 cko NPCs with or without Cyclopamine treatment for 48 h. Cells (5 × 10 5 ) are seeded initially. Data are shown as mean±s.e.m., t -test, ** P <0.01, n =3. ( g ) Confocal images of Tuj1 expression in the differentiated cells from in-vitro -cultured Rcor2 fl/fl and Rcor2 cko NPCs with or without Cyclopamine treatment. Tuj1 expressions are partially restored in Cyclopamine-treated Rcor2 cko cells. Scale bar, 20 μm. ( h ) Model of Rcor2 function in neurogenesis in the developing neocortex. Rcor2 safeguards cortical neurogenesis by recruiting LSD1 complex to the regulatory regions of Dlx2 and Shh genes, to inhibit the Shh pathway activation during development. The absence of Rcor2 leads to inhibition release of these genes and thus ectopic activation of Shh signalling in the developing neocortex, resulting in cortical neurogenesis defects. Full size image In addition, when adding Cyclopamine into the medium of the in-vitro -cultured NPCs for 48 h, the neurosphere sizes of Rcor2 cko NPCs were dramatically increased, similar in size to those of wild-type NPCs ( Fig. 7e ). Cell counting further confirmed about twofold increases in Rcor2 cko NPC numbers after Cyclopamine treatment compared with the untreated NPCs ( Fig. 7f ), suggesting improved proliferative ability of Rcor2 cko NPCs on Shh inhibition. Notably, ectopically activated Shh and Ptch1 signals in Rcor2 cko NPCs were downregulated and Dlx2 + cells decreased on Cyclopamine treatment ( Supplementary Fig. 8a ), indicating that Rcor2 regulates NPC proliferation through Shh signalling pathway. Depletion or knockdown of Rcor2 impairs neuronal differentiation of cortical RGCs during development ( Figs 2 , 3 and 5 , and Supplementary Figs 2, 3, 5 and 7 ). Hence, to further test whether the affected neuronal production caused by Rcor2 disruption can be rescued by Shh inhibition, Cyclopamine was introduced into the differentiation process of in-vitro -cultured NPCs. Immunostaining results showed the ratio of Tuj1 + cells in the Rcor2 cko group was significantly increased on Cyclopamine treatment, similar to those of the Rcor2 fl/fl group ( Fig. 7g and Supplementary Fig. 8b ), suggesting that the impaired neuronal differentiation of Rcor2-depleted NPCs could also be partially rescued by Shh inhibition in vitro . Histone demethylase LSD1/KDM1A can form complexes with different co-repressors in different cell types for fate regulation [42] , [43] , [44] . How specific subunits of LSD1 complex regulate gene activation and repression in brain development remains unclear. So far, three Rcor family genes ( Rcor1 / CoREST , Rcor2 and Rcor3 ) have been reported in mammalian genomes and their orthologous genes have also been found in Xenopus , Drosophilla and Caenorhabditis elegans [45] . Rcor1, as the first characterized Rcor family member, has been extensively investigated in previous reports. However, the roles of Rcor2 and testis-specific Rcor3 remain largely unknown. Using conditional knockout mouse models coupled with CRISPR/Cas9 genome-editing system, our study first identify that Rcor2 inhibits transcriptional activities by facilitating nucleosomal demethylase activities of LSD1 complex on the promoter regions of Dlx2 and Shh , both related to Shh signalling during cortical development. Furthermore, the ectopic activation of Shh signals caused by Rcor2 disruption results in inappropriate gene expression patterns in the developing dorsal neocortex and thus gives rise to defective NSC/NPC proliferation and differentiation, and finally severely impairs cortical neurogenesis and reduces brain size ( Fig. 7h ). As previously reported, Shh signalling pathway is essential to CNS development throughout different developmental stages for axes formation [10] , [46] , [47] . In the early developing telencephalon, Shh is mainly expressed in the MGE and PoA, to restrict ventral patterning and to maintain cortical interneuron progenitor identity, while maintaining a low level in the neural stem/progenitor cells and in mature neurons in the dorsal telencephalon [19] , [48] . In our study, we find that the LSD1 co-repressor Rcor2 is enriched in the core promoter regions of several genes downstream of Shh signalling such as Dlx2 , Dlx5 and Ascl1 , and the regulatory region of Shh ( Fig. 4h and Supplementary Fig. 4d ), thus sustaining the low activity of Shh signals during cortical development. In addition, not only the RNA transcripts but also the protein levels of the genes involved in Shh signalling is increased dramatically in the developing neocortex of Rcor2 cko brain in vivo and cultured Rcor2 cko NPCs in vitro ( Figs 5 and 6 , and Supplementary Fig. 6 ). This is the first evidence to demonstrate Rcor2 as a direct epigenetic regulator of Shh signalling pathway at the transcriptional level. Disrupting or depleting Rcor2 expression results in RGC division abnormality and cell death ( Fig. 2l,m ), resulting in reduction of newborn neuron population, neocortex thickness and brain size ( Figs 1f,g and 3a–e , and Supplementary Fig. 1d–g ). These neurogenesis defects could be partially rescued by inhibiting Shh signals ( Fig. 7 ), indicating that the ectopic Shh expression in the dorsal cortex could be a reason for defective cortical lamination on Rcor2 depletion, resulting in small brains. Interestingly, some research groups have considered that Shh is a mitogen regulating precursor cell proliferation in dorsal brain [15] , [18] . Studies from Shikata et al . [49] have suggested that strong upregulation of Shh signalling activates transition from dorsalized IPCs (Tbr2 + ) to ventralized IPCs (Dlx2 + ), whereas low expression of Shh is required for cortical IPC proliferation in VZ. Moreover, other findings revealed that Shh activation in dorsal cortex convert dorsal/ventral marker gene expression [50] . Consistent with that, our observations here suggested strong expression of Shh in dorsal brain on Rcor2 depletion, resulting in depletion of dorsalized NPCs/IPCs and reduction of pyramidal neurons. In addition, we found an increase of ventralized IPCs and interneurons in the developing neocortex. Combined with the previous studies discussed above, it is suggested that the temporal and spatial expression of Shh is critical for the elaborative regulation of neurogenesis. Rcor2 not only directly regulates transcription of Shh but also some other ventral marker genes, such as Dlx2 , Dlx5 and Ascl1 ( Fig. 4 and Supplementary Fig 4 ). GO analysis of RNA-seq and ChIP-seq did not reveal much direct bindings between Rcor2 and promoter regions of neuronal target genes, indicating that the neurogenesis defects and neuronal cell fate changes caused by Rcor2 depletion could be a systematic alteration of dorsal cell characteristics change and telencephalon environment disruption, in which Shh signalling might play a critical role as an effector. Consistent with this, RNA-seq analysis revealed that genes involved in cell migration, cell fate commitment and synapse organization were also changed on Rcor2 depletion, which could be results from the systematic alterations as well. However, we cannot rule out the direct role of Rcor2 in regulating synapse organization and circuits formation. Previous reports showed that ectopic Shh signalling in dorsal cortex induces expression of ventral marker genes and reduces expressions of dorsal marker genes [49] , [50] . Consistent with these observations, we found that when Shh signalling was abnormally activated on Rcor2 depletion in dorsal telencephalon at E13.5 and E15.5, the Shh receptor Ptch1 and its downstream ventral marker genes were dramatically upregulated, including Dlx2 , Nkx2.1 , Gsx2 , Ascl1 and so on ( Figs 5 , 6 and Supplementary Fig. 6 ). More importantly, we also found that expressions of dorsal marker genes such as Emx1/2 , Tbr2, Trnp1, Foxg1 and so on were reduced ( Fig. 5 and Supplementary Fig. 6 ). In addition, we observed increase of interneurons in dorsal neocortex ( Supplementary Fig 6c ), which could be generated locally due to ectopic expression of ventral genes. Taken together, our data support a model where Rcor2 directly represses transcription activities of Shh signalling pathway, to guarantee dorsal neocortex neurogenesis. Moreover, our in-vitro data recapitulated our in-vivo observations, highlighting the striking similarity of epigenetic regulation mechanisms both in vivo and in vitro . In summary, our findings open an avenue for the understanding of neurogenesis regulation via epigenetic regulatory complexes such as co-repressors in forebrain development. Aminals Adult Rcor2 LacZ mice (C57BL/6N-Rcor2 tm1a(EUCOMM)Wtsi ) were obtained from the Welcome Trust Sanger Institute Mouse Genetics Projects (Sanger MGP). Rcor2 fl/fl mice were generated by crossing Rcor2 LacZ mice with Rosa26 Flp mice. Rcor2 cko mice were produced by crossing Rcor2 fl/fl mice with Nestin Cre mice. Rcor2 fl/fl Emx1 Cre (Rcor2 Emx ) mice were generated by crossing Rcor2 fl/fl mice with Emx1 Cre mice. All mice had free access to food and water. All experiments were performed in accordance with the University of Health Guide for the Care and Use of Laboratory Animals and were approved by the Biological Research Ethics Committee of Tongji University. X-gal staining Embryos at E11.5 were perfused with 4% paraformaldehyde in PBS (pH 7.4) followed by staining with 1 g l −1 X-Gal (Invitrogen). Nissl staining and immunostaining of brain sections Embryos at the desired developmental stages were removed and transcardially perfused with ice-cold PBS (pH 7.4) followed by 4% paraformaldehyde in PBS (pH 7.4). Brains were dissected out and coronal sections were prepared using a vibratome (Leica Microsystems). For Nissl staining, brain slides were stained in 0.1% Cresyl violet for 3 min after dehydration and rehydration. Images were taken by Leica SCN400 (Leica Microsystems). For immunostaining, brain slides were subjected to antigen retrieval, followed by permeabilization (0.1% Triton X-100 in PBS), blocking (10% donkey serum in PBS) and antibody incubation. Images were acquired using a confocal laser scanning microscope (FV1000MPE-BX61WI, Olympus) and were analysed using FluoView (Olympus), Imaris (Bitplane) and Photoshop (Adobe Systems). Primary antibodies used were as follows: Rcor2 (1:50, catalogue number NBP1-74099, Novus Biological); Nes (1:300, catalogue number Rat-401, DSHB); Pax6 (1:100, DSHB); Sox2 (1:500, catalogue number sc-17319, Santa Cruz); BrdU (1:500, catalogue number ab6326, Abcam); Ki67 (1:300, catalogue number ab9260, Millipore); Satb2 (1:500, catalogue number ab34735, Abcam); Olig2 (1:200, catalogue number ab109186, Abcam); Shh (1:100, catalogue number sc-33943, Santa Cruz); Ptch1 (1:100, catalogue number sc-6149, Santa Cruz); Dlx2 (1:500, catalogue number ab117546, Abcam); Nkx2.1 (1:300, catalogue number ab76013, Abcam); Tbr1 (1:500, catalogue number ab31940, Abcam); Dcx (1:500, catalogue number ab18723, Abcam); Tbr2 (1:500, catalogue number ab23345, Abcam); Flag M2 (1:1,000, catalogue number F1804, Sigma); Map2 (1:500, catalogue number ab32454, Abcam); and Tuj1 (1:1,000, catalogue number mms-435p, Convance). Secondary antibodies used were as follows: goat or donkey anti-mouse or anti-rabbit Alexa-546-, Alexa-488- and Alexa-647-conjugated antibodies (1:500, Invitrogen). DNA was stained with 49,6-diamidino-2-phenylindole (1:10,000, catalogue number D1306, Invitrogen). Western blotting For western blotting analysis, cortical cells were lysed in lysis buffer (20 mM Tris pH 7.0, 1% Triton X-100, 0.5% NP-40, 250 mM NaCl, 3 mM EDTA and protease inhibitor cocktail). Proteins were separated by SDS–PAGE and transferred onto a nitrocellulose membrane. After membranes were blocked with 5% milk for 30 min, they were probed with various primary antibodies overnight at 4 °C, followed by incubation with secondary antibodies for 1 h at room temperature and visualized with enhanced chemiluminescence reagent (Thermo Scientific). Images have been cropped for presentation. Full-size images are presented in Supplementary Fig. 9 . cRNA probe synthesis and in situ hybridization cRNA probe was synthesized by forward primer 5′- GAGAGCCTCTGCCATCCA -3′ and reverse primer 5′- GCCAGAGAGATCCAGCCA -3′. For in situ hybridization, all operations were carried out under RNase-free conditions. Frozen sections of 20-μm thickness were hybridized with cRNA probes at a final concentration of 400 ng ml −1 overnight at 68 °C in hybridization solution (50% formamide, 10% dextran sulfate, 0.2% tRNA (Invitrogen), 1 × Denhardts solution (from a 50 × stock; Sigma), 1 × salt solution (containing 0.2 M NaCl, 0.01 M Tris, 5 mM NaH 2 PO 4 , 5 mM Na 2 HPO 4 , 5 mM EDTA pH 7.5)). After the sections were washed, alkaline phosphatase-coupled anti-digoxigenin Fab fragments were applied. For visualization of the labelled cRNAs, the sections were incubated in the dark in nitrobluetetrazolium/5-bromo-4-chloro-3-indolyl phosphate solution (Roche). Images were taken by Leica SCN400 (Leica Microsystems). Plasmid preparation and in-utero electroporation Rcor2 shRNA sequences were cloned into pSicoR-RFP vector, Rcor2 sequences were cloned into pMX-FLAG-HA-IRES-GFP vector and Shh shRNA sequences were cloned into pLL3.7 vector, as previously described [51] . In-utero electroporation was performed as previously described [51] . In brief, a timed pregnant CD-1 mouse or Rcor2 fl/fl mouse at E13.5 was anaesthetized, the uterine horns were exposed and 1 μl of plasmid DNA (1–3 μg μl −1 ) mixed with Fast Green (Sigma) was manually microinjected through the uterus into the lateral ventricle, using a beveled and calibrated glass micropipette (Drummond Scientific). For electroporation, five 50-ms pulses of 40–50 mV with a 950-ms interval were delivered across the uterus with two 9-mm electrode paddles positioned on either side of the head (ECM830, BTX). After the procedure, the uterus was placed back in the abdominal cavity and the wound was surgically sutured. The mouse was then placed in a 28 °C recovery incubator under close monitoring until it recovered and resumed normal activity. Related primer sequences were listed in Supplementary Table 1 . Time-lapse imaging of cortical slice culture Cortical slice cultures were prepared and time-lapse imaging was acquired as previously described [8] , [51] . About 1 day after in-utero electroporation, embryos were removed and the brain was extracted into ice-cold artificial cerebrospinal fluid containing the following: 125 mM NaCl, 5 mM KCl, 1.25 mM NaH 2 PO 4 , 1 mM MgSO 4 , 2 mM CaCl 2 , 25 mM NaHCO 3 , 20 mM glucose pH 7.4 and 310 mOsm l −1 . Brains were embedded in 3% low-melting agarose in artificial cerebrospinal fluid and sectioned at 400 mm using a vibratome (Leica Microsystems). Brain slices were transferred on to a slice culture insert (Millicell) in a glass-bottom Petri dish (MatTek Corporation) with culture medium containing (by volume): 66% Basal Medium Eagle (BME), 25% Hanks, 5% fetal bovine serum, 1% N2, 1% penicillin/streptomycin/glutamine (Invitrogen) and 0.66% D -(1)-glucose (Invitrogen). Cultures were maintained in a humidified incubator at 37 °C with constant 5% CO 2 supply. Twenty-four hours later, Petri dishes with slice cultures were transferred to an inverted microscope FV1000MPE-IX81ZDC (Olympus) and imaged every 20 min for about 2–3 days. Images were analysed by FluoView (Olympus), Imaris (Bitplane) and Photoshop (Adobe Systems). Reverse transcriptase–quantitative PCR Total RNAs of Rcor2 fl/fl and Rcor2 cko brains at desired developmental stages were extracted using TRIzol reagent (Invitrogen) according to the manufacturer’s instructions. Complementary DNA synthesis was performed with the M-MLV Reverse Transcriptase Kit (Promega) following the manufacturer’s instructions. Quantitative RT–PCR was performed using a SYBR Green Premix Ex Taq II (Takara) and signals were detected with ABI7500 Real-Time PCR System (Applied BioSystems). Related primer sequences were listed in Supplementary Table 1 and Gapdh was used as endogenous control. RNA-seq and data analysis For RNA-seq analysis, a timed pregnant Rcor2 fl/+ Nes Cre mouse crossed with Rcor2 fl/+ Nes Cre male mouse at E13.5 were anaesthetized. Embryos were removed separately and genotyping was performed to identify the Rcor2 fl/fl and Rcor2 cko pups. Cortical slices of Rcor2 fl/fl and Rcor2 cko embryos were prepared as described above. The VZ–SVZ regions were dissected separately and RNA was isolated using RNeasy Mini kit (Qiagen) according to the manufacturer’s instructions. RNA-seq was performed by Biodynamic Optical Imaging Center at Peking University. For data analysis, sequencing reads were mapped with default settings using Tophat software v2.0.3 to the mouse genome reference (UCSC mm9). Differential gene expression analysis and scatter plotting were performed with Cuffdiff and R as previously described [52] . ChIP-seq and ChIP–qPCR Rcor2 Flag mice were first generated by knocking in 3 × Flag sequences adjacent to the start codon ATG of Rcor2 gene locus by CRISPR/Cas9. Embryonic cortex were isolated from Rcor2 Flag and Rcor2 cko embryos at E13.5, respectively. Cross-linking, chromatin isolation, sonication and IP were performed using MAGnify Chromatin Immunoprecipitation System (Invitrogen) following the manufacturer’s instructions. Flag M2 antibody (1:1,000, catalogue number F1804, Sigma) and LSD1 antibody (1:1000, catalogue number 17721, Abcam) were used in the ChIP assays. Eluted DNA was used either for qPCR analysis as described above by using input DNA as the endogenous control or high-throughput sequencing. The pair-end sequencing was performed using Illumina Genome Analyzer IIx and Sequencing Kits (Version 5) after liabrary preparation. Illumina CASAVA pipeline v1.8.0 was used for the following sequence extraction and filtering. Accession codes: All sequencing-derived data reported in this study have been deposited in NCBI’s Gene Expression Omnibus (GEO) under accession number GSE75040 . How to cite this article : Wang, Y. et al . LSD1 co-repressor Rcor2 orchestrates neurogenesis in the developing mouse brain. Nat. Commun. 7:10481 doi: 10.1038/ncomms10481 (2016).